ERK phosphorylation and miR-181a expression modulate activation of human memory TH17 cells T helper (T H ) cell polarization during priming is modulated by a number of signals, but whether polarization to a given phenotype also influences recall responses of memory T H cells is relatively unknown. Here we show that miR-181a is selectively induced in both human and mouse naive T cells differentiating into the T H 17, but not T H 1 or T H 2 subset. In human memory T H 17 cells, miR-181a regulates responses to cognate antigens through modulation of ERK phosphorylation. By enhancing the signalling cascade from the T-cell receptor, such molecular network reduces the threshold of T H 17 cell activation. Moreover, at a late time point, the same network induces a self-regulatory mechanism dependent on ID3, a negative regulator of transcription factors that control RORC expression, thus modulating T H 17 activity. Our results demonstrate that the phenotype acquired by T H cells during priming contributes to their threshold of activation to secondary antigenic stimulations, thus influencing memory responses. Following antigenic stimulation, naive CD4 T cells proliferate and differentiate to a number of different memory and effector subsets, with responses tailored to the type of pathogen encountered, and able to migrate to specific tissues to eradicate infection. T H 17 cells are characterized by the ability to produce the proinflammatory cytokine IL-17, and are involved in epithelial and neutrophil-mediated immune responses against extracellular pathogens, especially bacteria and fungi. IL-17 induces the production of a broad range of proinflammatory cytokines and chemokines by a variety of cells [1] , and its expression must be carefully regulated. Indeed, despite their clear protective functions, T H 17 cells are also known to have prominent roles in the pathogenesis of autoimmune diseases such as rheumatoid arthritis and multiple sclerosis [2] . The differentiation of naive T cells into cytokine-producing effector T-cell subsets is influenced by a variety of factors, including the cytokine milieu and the presence of adequate co-stimulation, but also the affinity of the T-cell receptor (TCR) for the antigen, the duration of antigen stimulation, as well as the antigen concentration during priming [3] , [4] , [5] . For example, it is well established that mouse IL-4-producing T H 2 cells are preferentially generated by priming with a weak signal through the TCR while T H 1 cells are generated by priming with a strong signal [4] , [6] . More recently, low TCR strength was shown to promote IL-17 production by human CD4 T cells [7] . Among the factors implicated in the control of T-cell responses and TCR threshold of activation are microRNAs (miRNAs). MiRNAs are small noncoding RNA molecules with diverse and established roles in regulating differentiation, proliferation and function of most immune and non-immune cells investigated so far [8] , [9] . They also have critical roles in immune responses through their ability to modulate T-cell activation, proliferation and effector functions [9] . Two miRNAs were reported to be involved in the regulation of TCR activation: miR-146a and miR-181a (refs 9 , 10 , 11 , 12 , 13 ). MiR-146a regulates the intensity of NF-κB activation upon TCR stimulation. T cells lacking miR-146a are hyperreactive in both acute and chronic antigenic responses and give rise to defective memory responses [13] . MiR-181a is highly expressed in thymocytes [14] , and its dysregulated expression impairs both positive and negative thymic selection [11] . The effects of miR-181a during priming of naive T cells are mediated by the downregulation of a number of phosphatases, leading to increased levels of phosphorylated signalling intermediates, such as the extracellular signal-regulated kinases (ERK), and to an overall reduction of the TCR signalling threshold [11] . MiR-181a expression therefore increases responses to otherwise weak agonists and even antagonists, and is itself modulated by TCR signals [15] . Since all previous studies were focused on thymocyte development and priming of naive T cells, a role for miR-181a during a secondary T-cell response remains to be explored. Although most studies insofar were focused on the relationship between the properties of the input signals and their impact on polarization, the reciprocal interdependence between polarization and antigen responses is largely underexplored. Here, we show that human memory T H 17 cells differ from memory T H 1 and T H 2 cells because of their sustained ERK phosphorylation after the initial TCR triggering. Such sustained signalling depended on a feed-forward, self-maintaining loop involving miR-181a, which favoured the maintenance of ERK phosphorylation through the downmodulation of phosphatases. In turn, sustained ERK phosphorylation maintained high levels of miR-181a expression. This mechanism appeared to be predominant in T H 17 cells compared with other subsets, and enabled T H 17 cells to respond to anti-CD3 crosslinking or to specific antigens with a lower threshold of activation compared with T H 1 and T H 2 cells. Consistently, during priming of naive T cells, miR-181a was specifically induced by cytokines that favoured T H 17 but not T H 1 or T H 2 polarization. By inducing ID3, a negative regulator of transcription that acts by preventing binding of bHLH transcription factors to DNA, sustained ERK phosphorylation also regulated the expression of RORC and IL17 in recently activated T H 17 cells, thus limiting in a cell-intrinsic manner the potential negative consequences of T H 17-cell activation. Sustained ERK phosphorylation is therefore a characteristic feature of human memory T H 17 cells, which determines on one hand the threshold of activation to a subsequent encounter with an antigen and on the other hand it provides a built-in mechanism to dampen cytokine production after the initial response has occurred, thereby limiting potential tissue damage. Most importantly, our data provide the mechanistic bases for the observation that, given the same TCR specificity, the magnitude of a secondary response is also determined by the phenotype acquired during initial priming and polarization. miR-181a is acquired by differentiating T H 17 cells To study human memory T cells with a polarized T H 1, T H 2 and T H 17 phenotype, we isolated CD4 + CD45RA − T-cell subsets from the blood of healthy donors on the basis of the expression of CCR6, CXCR3 and CCR4, as previously described [16] . Memory T H 17 cells (CCR6 + CCR4 + ) isolated ex vivo expressed ~4-fold more miR-181a compared with T H 1 (CXCR3 + CCR6 − ) and T H 2 (CCR4 + CCR6 − ; Fig. 1a ), consistent with our previous findings using miRNA profiling [12] . On TCR stimulation, memory T H 17 cells further increased expression of miR-181a ( Fig. 1b ). 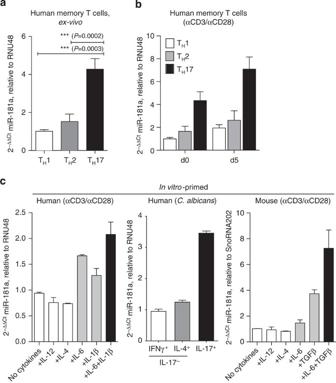Figure 1: miR-181a is highly expressed in TH17 cells. (a) Primary human memory TH1, TH2 and TH17 were sorted from peripheral blood of healthy donors on the basis of the expression of chemokine receptors and immediately lysed in Trizol for RNA extraction. Expression of miR-181a was assessed by qRT–PCR relative to RNU48, which was used as endogenous control. Shown are the compiled results from five independent donors (mean±s.d.).Pvalues were calculated by paired Student’st-test, two-tailed. (b) Primary human cell subsets were sorted from peripheral blood as inaand immediately lysed in Trizol or stimulated with plate-bound anti-CD3 (5 μg ml−1) and anti-CD28 (1 μg ml−1) antibodies for 5 days before lysis in Trizol. MiR-181a expression was assessed by qRT–PCR, using RNU48 as endogenous control. Shown are the compiled results from three independent donors (mean±s.d.). (c) (Left panel) Human naive T cells were stimulated with plate-bound anti-CD3 and anti-CD28 antibodies and cultured in the presence of the indicated cytokines for 12 days. Total RNA was then extracted and miR-181a expression measured by qRT–PCR. Shown are the compiled data for two donors (mean±s.e.m.). (Middle panel) Human naive CD4 T cells were sorted from the peripheral blood of healthy donors and labelled with CFSE, prior culture with autologous monocytes pulsed with heat-inactivatedC. albicans. The proliferating T cells were expanded with IL-2, and CFSE-negative antigen-specific cells were analysed on day 17 for the production of IL-17, IL-4 and IFN-γ by intracellular staining. T cells expressing the signature cytokines IFN-γ, IL-4 and IL-17 were sorted by cytokine secretion assay and lysed in Trizol before analysis of miR-181a expression. Data are representative of two independent experiments. (Right panel) Mouse naive 2D2 cells were isolated from spleen and lymph nodes and were stimulated with plate-bound anti-CD3 and anti-CD28 antibodies in the presence of the indicated cytokines. Polarization was assessed by intracellular staining 5 days later and miR-181a expression was assessed by qRT–PCR; snoRNA202 was used as endogenous control. Shown are the compiled data for three mice (mean±s.e.m.), representative of five independent experiments. Figure 1: miR-181a is highly expressed in T H 17 cells. ( a ) Primary human memory T H 1, T H 2 and T H 17 were sorted from peripheral blood of healthy donors on the basis of the expression of chemokine receptors and immediately lysed in Trizol for RNA extraction. Expression of miR-181a was assessed by qRT–PCR relative to RNU48, which was used as endogenous control. Shown are the compiled results from five independent donors (mean±s.d.). P values were calculated by paired Student’s t -test, two-tailed. ( b ) Primary human cell subsets were sorted from peripheral blood as in a and immediately lysed in Trizol or stimulated with plate-bound anti-CD3 (5 μg ml −1 ) and anti-CD28 (1 μg ml −1 ) antibodies for 5 days before lysis in Trizol. MiR-181a expression was assessed by qRT–PCR, using RNU48 as endogenous control. Shown are the compiled results from three independent donors (mean±s.d.). ( c ) (Left panel) Human naive T cells were stimulated with plate-bound anti-CD3 and anti-CD28 antibodies and cultured in the presence of the indicated cytokines for 12 days. Total RNA was then extracted and miR-181a expression measured by qRT–PCR. Shown are the compiled data for two donors (mean±s.e.m.). (Middle panel) Human naive CD4 T cells were sorted from the peripheral blood of healthy donors and labelled with CFSE, prior culture with autologous monocytes pulsed with heat-inactivated C. albicans . The proliferating T cells were expanded with IL-2, and CFSE-negative antigen-specific cells were analysed on day 17 for the production of IL-17, IL-4 and IFN-γ by intracellular staining. T cells expressing the signature cytokines IFN-γ, IL-4 and IL-17 were sorted by cytokine secretion assay and lysed in Trizol before analysis of miR-181a expression. Data are representative of two independent experiments. (Right panel) Mouse naive 2D2 cells were isolated from spleen and lymph nodes and were stimulated with plate-bound anti-CD3 and anti-CD28 antibodies in the presence of the indicated cytokines. Polarization was assessed by intracellular staining 5 days later and miR-181a expression was assessed by qRT–PCR; snoRNA202 was used as endogenous control. Shown are the compiled data for three mice (mean±s.e.m. ), representative of five independent experiments. Full size image To ask whether the preferential expression of miR-181a was imprinted at the time of priming, we sorted human naive CD4 T cells and we activated them in vitro with anti-CD3 and anti-CD28 antibodies in the presence of polarizing cytokines. Addition of IL-12 or IL-4 (for T H 1 and T H 2 differentiation, respectively) had no effect on miR-181a expression, whereas miR-181a was induced by signals that favour human T H 17 cell differentiation [17] , namely IL-6+IL-1β ( Fig. 1c , left panel). Interestingly, addition of the individual cytokines (IL-6 or IL-1β) was also able to induce moderate expression of miR-181a, suggesting that cytokine signalling upon priming is sufficient to induce miR-181a expression in T H 17-polarizing conditions. Human naive CD4 T cells were also in vitro primed in the presence of Candida albicans as described [18] . In these conditions, T cells acquired a mixed phenotype ( Supplementary Fig. 1 ), and a cytokine secretion assay was therefore used to separate IL-17 – (IFN-γ + or IL-4 + ) and IL-17 + cells from the same culture. Consistent with the findings on memory T H 17 cells isolated directly from the peripheral blood, also these in vitro -polarized IL-17-producing cells expressed higher levels of miR-181a compared with the non-IL-17-producing T cells ( Fig. 1c , middle panel). Finally, addition of T H 17-polarizing cytokines (IL-6 and TGFβ) alone or in combination, to mouse naive T cells primed in vitro with antibodies to CD3 and CD28 also induced higher levels of miR-181a compared with the addition of IL-12 or IL-4, respectively ( Fig. 1c , right panel). Collectively, these data indicate that miR-181a is acquired by both human and mouse naive T cells differentiating towards the T H 17 lineage, and uncover an important role for cytokine signalling in its induction. miR-181a contributes to sustained ERK phosphorylation MiR-181a was shown to be highly expressed in thymocytes and to regulate the threshold of activation of these cells by modulating TCR signalling through ERK phosphorylation [11] , [14] . We therefore asked whether memory T H 17 cells display differences in the threshold of activation as compared with memory T H 1 and T H 2 cells. T H -cell subsets were isolated ex vivo from peripheral blood and stimulated with increasing concentrations of anti-CD3 antibody together with a fixed amount of plate-bound anti-CD28 antibody. Five days after stimulation, cell proliferation in each subset was assessed by 3 H-thymidine incorporation assay ( Fig. 2a ). At low concentrations of anti-CD3, a proliferative response was detectable only in memory T H 17 cells, indicating that this subset has the lowest threshold of activation. With increasing concentrations, proliferation of T H 17 cells was comparable to that of memory T H 1 cells, but remained superior to that of memory T H 2 cells, which responded only at relatively high anti-CD3 concentrations. Consistently, EC 50 values calculated on seven independent donors were significantly lower in T H 17 cells as compared with T H 2 and T H 1 cells ( Fig. 2b ). 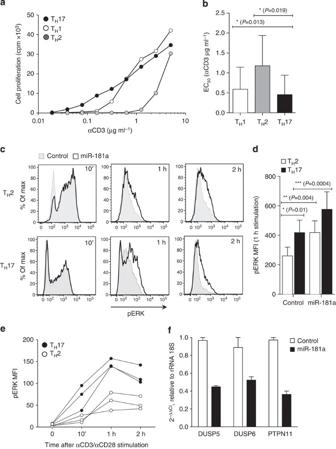Figure 2: Increased ERK phosphorylation mediated by miR-181a. (a) Primary human memory TH1, TH2 and TH17 were sorted from peripheral blood and immediately stimulated on plate-bound anti-CD28 (1 μg ml−1) with increasing concentrations of anti-CD3 antibody. Five days after stimulation, cell proliferation was assessed by3H-thymidine incorporation assay. One representative donor is shown. (b) Compiled EC50values calculated for seven independent donors analysed as ina(mean±s.d.).Pvalues were calculated by paired Student’st-test, two-tailed. (c) TH2 and TH17 cells were sorted from peripheral blood and immediately transfected with a miR-181a mimic or a negative scrambled control oligonucleotide. Forty-eight hours after transfection, cells were stimulated with anti-CD3 and anti-CD28 antibodies for the indicated times and phosphorylation of ERK was assessed by intracellular staining. Shown are data from one representative donor. (d) Compiled results of multiple experiments as inc(n=4 individual donors for TH2 andn=6 individual donors for TH17 (mean±s.d.).Pvalues were calculated by paired (within each subset) or unpaired (across different T-cell subsets) Student’st-test, two-tailed. Shown are MFIs for pERK observed after 1 h of stimulation with anti-CD3 and anti-CD28 antibodies. (e) Human TH17 and TH2 clones were stimulated with 1 μg ml−1anti-CD28 and 5 μg ml−1of anti-CD3 antibodies. Levels of ERK phosphorylation were measured at the indicated times by intracellular staining. Each line represents one clone. (f) TH17 cells were transfected as inc, and total RNA was extracted to assess expression of the indicated phosphatases by qRT–PCR. 18S RNA was used as endogenous control. Data are representative of two independent experiments. Figure 2: Increased ERK phosphorylation mediated by miR-181a. ( a ) Primary human memory T H 1, T H 2 and T H 17 were sorted from peripheral blood and immediately stimulated on plate-bound anti-CD28 (1 μg ml −1 ) with increasing concentrations of anti-CD3 antibody. Five days after stimulation, cell proliferation was assessed by 3 H-thymidine incorporation assay. One representative donor is shown. ( b ) Compiled EC 50 values calculated for seven independent donors analysed as in a (mean±s.d.). P values were calculated by paired Student’s t -test, two-tailed. ( c ) T H 2 and T H 17 cells were sorted from peripheral blood and immediately transfected with a miR-181a mimic or a negative scrambled control oligonucleotide. Forty-eight hours after transfection, cells were stimulated with anti-CD3 and anti-CD28 antibodies for the indicated times and phosphorylation of ERK was assessed by intracellular staining. Shown are data from one representative donor. ( d ) Compiled results of multiple experiments as in c ( n =4 individual donors for T H 2 and n =6 individual donors for T H 17 (mean±s.d.). P values were calculated by paired (within each subset) or unpaired (across different T-cell subsets) Student’s t -test, two-tailed. Shown are MFIs for pERK observed after 1 h of stimulation with anti-CD3 and anti-CD28 antibodies. ( e ) Human T H 17 and T H 2 clones were stimulated with 1 μg ml −1 anti-CD28 and 5 μg ml −1 of anti-CD3 antibodies. Levels of ERK phosphorylation were measured at the indicated times by intracellular staining. Each line represents one clone. ( f ) T H 17 cells were transfected as in c , and total RNA was extracted to assess expression of the indicated phosphatases by qRT–PCR. 18S RNA was used as endogenous control. Data are representative of two independent experiments. Full size image The difference in the threshold of activation in particular between T H 17 and T H 2 cells prompted us to investigate whether miR-181a could modulate ERK phosphorylation induced by TCR triggering in these cells. Memory T H 17 and T H 2 cells were transfected with either a miR-181a mimic or a scrambled control oligonucleotide and then stimulated with anti-CD3 and anti-CD28 antibodies. ERK phosphorylation was assessed by intracellular staining ( Fig. 2c ). Compared with T H 2 cells, T H 17 cells showed moderately but consistently higher levels of ERK phosphorylation after 1 h of stimulation ( Fig. 2d ). Overexpression of miR-181a mimic allowed sustained ERK phosphorylation for a longer period of time in both T-cell subsets ( Fig. 2c,d ), suggesting that levels of ERK phosphorylation in memory T cells may be regulated by miR-181a expression regardless of their phenotype. The ability of miR-181a to regulate ERK phosphorylation implies that the higher endogenous levels of miR-181a observed specifically in T H 17 cells may lead to sustained ERK phosphorylation compared with other T-cell subsets. We therefore isolated T H 17 and T H 2 clones from memory T cells by limiting dilution. Increased and sustained ERK phosphorylation was observed upon stimulation of all analysed clones, although T H 17 cells showed consistently higher levels ( Fig. 2e ). Remarkably, T H 17 clones maintained ERK phosphorylation for a very prolonged period of time (up to 5 days) after stimulation ( Supplementary Fig. 2 ). The link between miR-181a expression and modulation of ERK phosphorylation through the regulation of phosphatases is well established in a number of experimental systems [11] , [15] , [19] , [20] , [21] , [22] . We therefore analysed the expression of DUSP5 and DUSP6, two ERK-specific phosphatases acting in the nucleus and cytoplasm, respectively [23] , and also of the phosphatase PTPN11 (SHP-2), which are all validated direct targets of miR-181a (ref. 11 ). Consistent with previous work [11] , forced miR-181a expression in ex vivo -isolated memory T H 17 cells led to a reduction in the mRNA levels of all of these phosphatases ( Fig. 2f ), indicating that miR-181a expression in T H 17 cells might lead to sustained ERK phosphorylation through the downregulation of phosphatases that negatively control TCR signalling. miR-181a modulates antigen sensitivity in T H 17 cells We next assessed whether miR-181a expression could modulate the proliferative responses of T H 17 cells to antigens presented by antigen-presenting cells. Human memory T H 17 cells were isolated from peripheral blood, labelled with CFSE (5(6)-carboxyfluorescein diacetate N-hydroxysuccinimidyl ester) and cultured with C. albicans in the presence of autologous monocytes. In this experimental system, T-cell proliferation depends on MHC-II antigen presentation [18] , [24] . After expansion in IL-2, the specific proliferating blast cells were first transfected with a miR-181a mimic, a scrambled control oligonucleotide or a blocking miR-181a antagomir, and then restimulated with monocytes in the presence of increasing concentrations of C. albicans antigens. Forced expression of miR-181a led to a more robust proliferation of memory T H 17 cells in low stimulatory conditions ( Fig. 3a ). Importantly, blocking miR-181a in T H 17 cells using an antagomir led to reduced activation and proliferation of these cells ( Fig. 3a ). Similar results were obtained transfecting ex vivo freshly isolated T H 17 cells and then stimulating them with different numbers of C. albicans particles ( Fig. 3b ). Similar results were also obtained using a completely different antigen, the tetanus toxoid ( Supplementary Fig. 3 ). Collectively, these data indicate that miR-181a expression regulates T-cell proliferation in response to cognate antigenic stimulation. 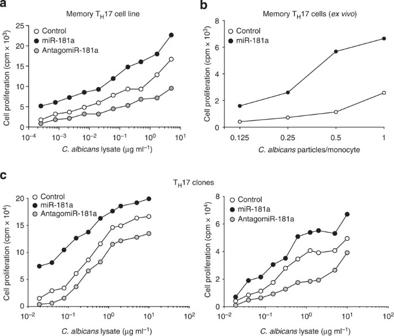Figure 3: miR-181a modulates TH17-cell activation and proliferation. (a) Primary TH17 cells were sorted from peripheral blood, loaded with CFSE and stimulated with autologous monocytes in the presence ofC. albicans. Five days after stimulation, antigen-specific cells (CFSElo) were recovered by sorting, divided into three aliquots and transfected with either a scrambled control, a miR-181a mimic or a blocking miR-181a antagomir. Forty-eight hours after transfection, cells were restimulated with autologous monocytes and increasing concentrations ofC. albicanslysate, and proliferation was assessed 4 days later by3H-thymidine incorporation assay. (b) Primary TH17 cells were sorted from peripheral blood and immediately divided into two aliquots transfected with either a scrambled control or a miR-181a mimic. Forty-eight hours post transfection, cells were stimulated with irradiated autologous monocytes pulsed with increasing numbers of wholeC. albicansparticles. Cell proliferation was measured after 72 h of stimulation by3H-thymidine incorporation assay. (c) Cells were treated as inaexcept thatC. albicans-specific CFSElocells were individually cloned, each clone was expanded, divided into three aliquots and transfected with either a scrambled control, a miR-181a mimic or antagomir before restimulation with increasing numbers of autologous monocytes pulsed withC. albicans. Proliferation was assessed 3 days after by3H-thymidine incorporation assay. Two representative clones are shown. Figure 3: miR-181a modulates T H 17-cell activation and proliferation. ( a ) Primary T H 17 cells were sorted from peripheral blood, loaded with CFSE and stimulated with autologous monocytes in the presence of C. albicans . Five days after stimulation, antigen-specific cells (CFSE lo ) were recovered by sorting, divided into three aliquots and transfected with either a scrambled control, a miR-181a mimic or a blocking miR-181a antagomir. Forty-eight hours after transfection, cells were restimulated with autologous monocytes and increasing concentrations of C. albicans lysate, and proliferation was assessed 4 days later by 3 H-thymidine incorporation assay. ( b ) Primary T H 17 cells were sorted from peripheral blood and immediately divided into two aliquots transfected with either a scrambled control or a miR-181a mimic. Forty-eight hours post transfection, cells were stimulated with irradiated autologous monocytes pulsed with increasing numbers of whole C. albicans particles. Cell proliferation was measured after 72 h of stimulation by 3 H-thymidine incorporation assay. ( c ) Cells were treated as in a except that C. albicans -specific CFSE lo cells were individually cloned, each clone was expanded, divided into three aliquots and transfected with either a scrambled control, a miR-181a mimic or antagomir before restimulation with increasing numbers of autologous monocytes pulsed with C. albicans . Proliferation was assessed 3 days after by 3 H-thymidine incorporation assay. Two representative clones are shown. Full size image Since in the above experiments we utilized memory T H 17 cells containing a pool of different TCR specificities, the possibility remained that altered miR-181a expression was somehow favoring the expansion of a few selected clones. To assess whether increased miR-181a expression leads to a cell-intrinsic decrease in the threshold of activation to a given antigen, we selected individual T H 17 clones specific for C. albicans. Each clone (composed of cells carrying the same TCR specificity) was then divided into aliquots and transfected with either a miR-181a mimic, antagomir or a control oligonucleotide. As shown in Fig. 3c for two exemplary T-cell clones, cells transfected with a miR-181a mimic or antagomir showed increased or decreased proliferation, respectively, in response to stimulation with C. albicans , as compared with the same cells transfected with a control oligonucleotide. These data indicate that, through the regulation of ERK phosphorylation, miR-181a modulates antigen sensitivity in T H 17 cells in a cell-intrinsic manner. Increased sensitivity of antigen-specific T H 17 cells Our data imply that if a given antigen is recognized by two memory T cells with the same TCR specificity, their proliferative response will also be dictated in a cell-intrinsic manner by the phenotype acquired during the initial priming. Since also mouse T H 17 cells expressed higher levels of miR-181a compared with other T-cell subsets ( Fig. 1c ), to address more specifically this possibility in an in vivo system, we took advantage of TCR-transgenic murine cells. MOG (myelin oligodendrocyte glycoprotein)-specific 2D2 cells [25] were adoptively transferred into C57Bl/6 mice. Immunization was then performed with MOG 35–55 in the presence of either complete Freund’s adjuvant (CFA), which favoured differentiation mainly of IL-17-producing T cells, or alum, which instead favoured polarization of IL-4-producing T cells ( Fig. 4a ). Six days after immunization, polarized 2D2 cells were recovered from the draining lymph nodes and restimulated in vitro with dendritic cells pulsed with increasing concentration of MOG 35–55 . Proliferation was assessed by a 3 H-thymidine incorporation assay 3 days later. Similar to human cells stimulated with anti-CD3 and anti-CD28 antibodies, in vivo -polarized 2D2 transgenic T H 17 cells proliferated much more vigorously and at lower concentrations of antigen compared with T H 2 cells expressing an identical TCR ( Fig. 4b ). 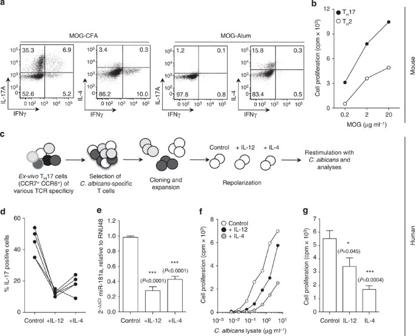Figure 4: Low threshold of TCR activation in TH17 cells. (a) Transgenic mouse 2D2 naive T cells were adoptively transferred into C57Bl/6 wild-type recipients (105cells per mouse) and polarizedin vivowith MOG35–55and either complete Freund’s adjuvant or alum as adjuvants. Six days after, challenge cells were recovered from the draining lymph nodes and their polarization assessed by intracellular cytokine staining after restimulation with PMA and ionomycin for 5 h. Data are representative of three independent experiments. (b) Cells as inawere recovered from the draining lymph nodes after adoptive transfer andin vivopolarization, and were restimulatedin vitrowith bone marrow-derived dendritic cells matured overnight with lipopolysaccharide and pulsed with increasing concentrations of MOG35–55peptide. Cell proliferation was assessed after 3 days by3H-thymidine incorporation assay. Fifteen mice were pooled for the TH17 conditions (complete Freund’s adjuvant) and thirty for TH2 (alum). Representative of two independent experiments. (c) Schematic representation of the experimental setup for panelsd–g:C. albicans-specific central memory human TH17 cells were selected from the total pool of TH17 cells, and individual cells were cloned and expanded. Each clone was divided into three aliquots that were cultured under either non-polarizing conditions (control) or with addition of IL-12 or IL-4. (d) Percentage of IL-17-producing cells in individual clones was assessed by stimulation with PMA and ionomycin and intracellular staining. Each dot represents one clone and subclones are connected by lines. (e) miR-181a expression was assessed in the same five clones as ind. Shown are the compiled results for all the clones (mean±s.e.m.).Pvalues were calculated by paired Student’st-test, two-tailed. (f) The same clones as indwere restimulated with increasing concentrations ofC. albicanslysate in the presence of autologous monocytes. Three days after stimulation, T-cell proliferation was assessed by3H-thymidine incorporation assay. One representative clone is shown. (g) Overall proliferation of five clones treated as infand stimulated with 1.6 μg ml−1ofC. albicanslysate (mean±s.e.m.).Pvalues were calculated by paired Student’st-test, two-tailed. Figure 4: Low threshold of TCR activation in T H 17 cells. ( a ) Transgenic mouse 2D2 naive T cells were adoptively transferred into C57Bl/6 wild-type recipients (10 5 cells per mouse) and polarized in vivo with MOG 35–55 and either complete Freund’s adjuvant or alum as adjuvants. Six days after, challenge cells were recovered from the draining lymph nodes and their polarization assessed by intracellular cytokine staining after restimulation with PMA and ionomycin for 5 h. Data are representative of three independent experiments. ( b ) Cells as in a were recovered from the draining lymph nodes after adoptive transfer and in vivo polarization, and were restimulated in vitro with bone marrow-derived dendritic cells matured overnight with lipopolysaccharide and pulsed with increasing concentrations of MOG 35–55 peptide. Cell proliferation was assessed after 3 days by 3 H-thymidine incorporation assay. Fifteen mice were pooled for the T H 17 conditions (complete Freund’s adjuvant) and thirty for T H 2 (alum). Representative of two independent experiments. ( c ) Schematic representation of the experimental setup for panels d – g : C. albicans -specific central memory human T H 17 cells were selected from the total pool of T H 17 cells, and individual cells were cloned and expanded. Each clone was divided into three aliquots that were cultured under either non-polarizing conditions (control) or with addition of IL-12 or IL-4. ( d ) Percentage of IL-17-producing cells in individual clones was assessed by stimulation with PMA and ionomycin and intracellular staining. Each dot represents one clone and subclones are connected by lines. ( e ) miR-181a expression was assessed in the same five clones as in d . Shown are the compiled results for all the clones (mean±s.e.m.). P values were calculated by paired Student’s t -test, two-tailed. ( f ) The same clones as in d were restimulated with increasing concentrations of C. albicans lysate in the presence of autologous monocytes. Three days after stimulation, T-cell proliferation was assessed by 3 H-thymidine incorporation assay. One representative clone is shown. ( g ) Overall proliferation of five clones treated as in f and stimulated with 1.6 μg ml −1 of C. albicans lysate (mean±s.e.m.). P values were calculated by paired Student’s t -test, two-tailed. Full size image To be able to assess responses of primary human T H 1, T H 2 and T H 17 cells bearing an identical TCR specificity, we exploited human T-cell plasticity, namely the ability of the cells to be at least in part repolarized under specific in vitro culture conditions [26] . T-cell clones were generated by limiting dilution from CCR7 + CCR6 + CCR4 + memory T cells. At the time of expansion, each clone was divided into three aliquots that were cultured under either non-polarizing conditions (control) or in the presence of IL-12 (‘T H 1-like’ conditions) or IL-4 (‘T H 2-like’ conditions; schematic in Fig. 4c ). T-cell clones cultured under non-polarizing conditions were mainly producing IL-17, consistent with the notion that a high frequency of memory T cells specific for C. albicans are T H 17. Treatment of the same clones with IL-4 and IL-12 had as a predominant effect the loss of the T H 17 phenotype (as determined by the reduction in IL-17 production) and, notably, a concomitant loss in miR-181a expression ( Fig. 4d,e ). Culture of the same clones with IL-12 or IL-4 led to a mild upregulation of IFNγ and IL-4, respectively ( Supplementary Fig. 4 ), indicating loss of the T H 17 phenotype together with some degree of repolarization. Paired T-cell clones were then compared for their capacity to proliferate in response to increasing concentrations of C. albicans antigens in the presence of autologous monocytes. T-cell clones cultured in the presence of IL-12 or IL-4 showed overall reduced responses compared with the same T H 17 cells cultured in the absence of repolarizing cytokines, especially in the presence of IL-4 ( Fig. 4f,g ). These data indicate that differences in proliferating capacity are intrinsic to the phenotype of the responding T cells. To further strengthen our data, we were able to isolate from the blood of a healthy donor memory T-cell clones specific for C. albicans and carrying identical Vβ CDR3 TCR sequences, but with different phenotypes (namely T H 17 and T H 2; ref. 27 ). On restimulation of these clones with C. albicans lysates, T H 17 cells proliferated more vigorously compared with T H 2 cells expressing the same Vβ TCR specificity ( Supplementary Fig. 5a ). Importantly, the magnitude of proliferation closely correlated with the levels of expression of miR-181a in each individual clone, with the T H 17 clone that displayed the strongest proliferation also showing the highest expression of this miRNA ( Supplementary Fig. 5b ). On the whole, our data indicate that T H 17 cells, independently of TCR specificity, have an intrinsically lower threshold of activation to cognate antigens compared with other subsets such as T H 2. Moreover, such threshold is at least in part regulated by sustained ERK phosphorylation and miR-181a expression. ID3 is induced upon activation in an ERK-dependent manner As mentioned above, T H 17 clones showed sustained ERK phosphorylation for prolonged periods of time, as compared with T H 2 clones ( Supplementary Fig. 2 ). Specifically, by analysing a broad panel of phosphorylated proteins, we found that at late time points (day 5), the majority of signalling molecules did not show any significant change compared with baseline (day 0) in both T H 17 and T H 2 cells, consistent with the notion that most of these pathways have early and transient kinetics. However, we found some sustained STAT protein phosphorylation, which was somewhat expected on T-cell stimulation, as it was previously shown that STAT3 and STAT5 contribute to regulate IL-17 production and RORC expression [18] , [28] , [29] , [30] , [31] . Most importantly, we found that ERK1/2 remained phosphorylated in T H 17 (but not in T H 2) cells at more than 4-fold over the baseline after 5 days from the initial stimulation ( Supplementary Fig. 2 ). Increased ERK phosphorylation in activated T H 17 clones compared with T H 2 was also confirmed by intracellular staining ( Fig. 5a,b ). Since human memory T H 17 cells transiently lose the ability to produce IL-17 5 days after antigenic stimulation ( Fig. 5c ) [18] , and since ERK phosphorylation was sustained in T H 17 cells within the same time frame, we assessed whether loss of cytokine production by T H 17 cells was also dependent on ERK signalling. First, we established working concentrations of a specific ERK inhibitor (ERKi) that did not completely block TCR signalling, but still allowed T-cell activation and proliferation as assessed by CFSE dilution ( Fig. 5d ). T H 17 clones were either left resting or stimulated with anti-CD3 and anti-CD28 antibodies in the presence or absence of increasing concentrations of ERKi. After 5 days, the percentage of IL-17-producing cells was assessed by intracellular staining. Although the majority of cells lost the ability to express IL-17 after stimulation, cytokine production was almost completely recovered with increasing concentrations of ERKi ( Fig. 5e ). In these same experimental conditions, both IL17 and RORC mRNA expression were almost completely recovered in the presence of ERKi ( Fig. 5f ). 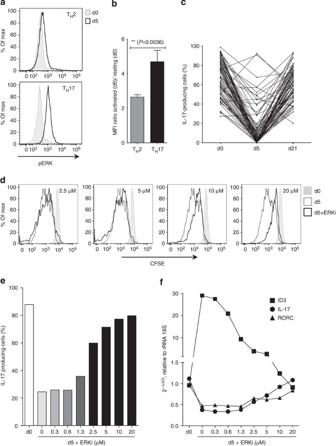Figure 5: Transient loss of IL-17 expression depends on ERK signalling. (a,b) TH17 and TH2 clones were either left resting (d0) or were stimulated with plate-bound anti-CD3 and anti-CD28 antibodies for 5 days, and ERK phosphorylation (pERK) was assessed by intracellular staining. Shown inais one representative staining, whilebshows the mean fluorescence intensity (MFI) for 30 independent clones (mean±s.e.m.).Pvalues were calculated by unpaired Student’st-test, two-tailed. (c) Primary human memory TH17 cells were sortedex vivofrom peripheral blood and cloned. T-cell clones were either left resting, or were stimulated with plate-bound anti-CD3 and anti-CD28 antibodies for 5 and 21 days. At each time point, cells were restimulated with PMA and ionomycin for 5 h for intracellular cytokine staining to assess cytokine production. Each line represents one individual clone. (d) Human TH17 clones were loaded with CFSE before stimulation with plate-bound anti-CD3 and anti-CD28 antibodies in the presence or absence of increasing concentration of ERKi. Proliferation was assessed 5 days later on the basis of CFSE dilution. Representative of three independent experiments. (e) Cells were treated as ind, except that IL-17 production was assessed by intracellular staining. (f) Cells were treated as ind, except that total RNA was extracted to assess expression ofRORC, IL17andID3mRNA. rRNA 18S was used as endogenous control. Data are representative of three independent experiments. Figure 5: Transient loss of IL-17 expression depends on ERK signalling. ( a , b ) T H 17 and T H 2 clones were either left resting (d0) or were stimulated with plate-bound anti-CD3 and anti-CD28 antibodies for 5 days, and ERK phosphorylation (pERK) was assessed by intracellular staining. Shown in a is one representative staining, while b shows the mean fluorescence intensity (MFI) for 30 independent clones (mean±s.e.m.). P values were calculated by unpaired Student’s t -test, two-tailed. ( c ) Primary human memory T H 17 cells were sorted ex vivo from peripheral blood and cloned. T-cell clones were either left resting, or were stimulated with plate-bound anti-CD3 and anti-CD28 antibodies for 5 and 21 days. At each time point, cells were restimulated with PMA and ionomycin for 5 h for intracellular cytokine staining to assess cytokine production. Each line represents one individual clone. ( d ) Human T H 17 clones were loaded with CFSE before stimulation with plate-bound anti-CD3 and anti-CD28 antibodies in the presence or absence of increasing concentration of ERKi. Proliferation was assessed 5 days later on the basis of CFSE dilution. Representative of three independent experiments. ( e ) Cells were treated as in d , except that IL-17 production was assessed by intracellular staining. ( f ) Cells were treated as in d , except that total RNA was extracted to assess expression of RORC, IL17 and ID3 mRNA. rRNA 18S was used as endogenous control. Data are representative of three independent experiments. Full size image We previously showed that loss of IL17 transcription in activated T cells was due, at least in part, to a loss in RORγt expression [18] . Here we hypothesized that ERK-dependent induction of a negative regulator of transcription may also have a role in the loss of RORC mRNA expression. The region upstream the RORC transcription start site was shown to contain several binding sites for the bHLH protein E2A (ref. 32 ). ID3, a negative regulator of bHLH protein activity, was shown to mildly influence INFγ expression [33] and to counteract IL-17 production and T H 17 differentiation in the mouse [34] . Moreover, ID3 expression was also shown to depend on ERK activation in T cells [35] . We therefore investigated the expression of ID3 upon TCR stimulation. Interestingly, ID3 expression inversely correlated with RORC and IL17 expression in activated T H 17 cells, with a strong induction 5 days after initial stimulation ( Fig. 5f ). ID3 induction was also dependent on ERK phosphorylation, as assessed by activating cells in the presence of ERKi ( Fig. 5f ). These data point towards a direct role for ID3 as a negative regulator of RORC (and IL17 ) expression in recently activated T H 17. ID3 inhibits RORC and IL17 expression To investigate expression and function of ID3 in this system, we stimulated freshly isolated T H 17 cells with plate-bound anti-CD3 and anti-CD28, and assessed the expression of RORC and ID3 mRNA over time ( Fig. 6a ). RORC expression showed a strong downregulation in the first 6 days after stimulation, which was slowly recovered over time and correlated with the transient downregulation of IL-17 expression that we previously described ( Fig. 5c ). Vice versa, ID3 expression showed an opposite trend, with increased expression that slowly returned to low, baseline levels ( Fig. 6a ). Similar results were obtained using antigen-specific T H 17-cell clones stimulated with Mycobacterium tuberculosis , which upon restimulation showed increased ID3 expression and concomitant loss of RORC and IL17 mRNA ( Fig. 6b ). 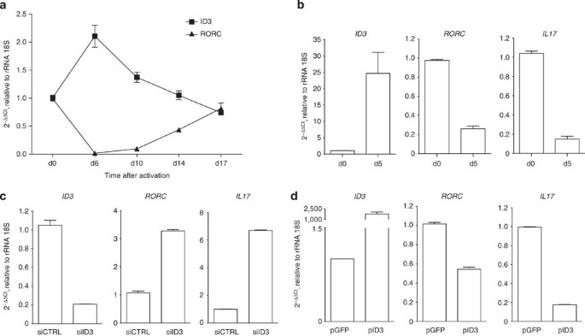Figure 6: ID3 repressesRORCandIL-17expression. (a)Ex vivo-isolated TH17 cells were either left resting or were stimulated with plate-bound anti-CD3 and anti-CD28 antibodies and expanded for up to 17 days. At the indicated time points, total RNA was extracted and expression ofRORCandID3was assessed by qRT–PCR. Representative of two independent experiments. (b) Individual TH17 clones specific forM. tuberculosiswere either left resting or were restimulated with plate-bound anti-CD3 and anti-CD28 antibodies for 5 days, after which expression ofID3,RORCandIL17was measured by qRT–PCR. Shown are the compiled data of six independent clones, representative of two independent experiments. (c) TH17 cells were sortedex vivoand transfected with a siRNA against ID3 (siID3) or a negative control (siCTRL). Cells were allowed to recover for 48 h before stimulation with anti-CD3 and anti-CD28 antibodies for another 48 h hours, after which expression ofID3,RORCandIL17was measured by qRT–PCR. Representative of at least three independent experiments. (d)Ex vivo-isolated TH17 cells were transfected with a plasmid to force expression of ID3 or with a control plasmid expressing only GFP. Forty-eight hours after transfection, total RNA was extracted and levels ofID3,RORCandIL17were assessed by qRT–PCR. Data are representative of at least three independent experiments. Figure 6: ID3 represses RORC and IL-17 expression. ( a ) Ex vivo -isolated T H 17 cells were either left resting or were stimulated with plate-bound anti-CD3 and anti-CD28 antibodies and expanded for up to 17 days. At the indicated time points, total RNA was extracted and expression of RORC and ID3 was assessed by qRT–PCR. Representative of two independent experiments. ( b ) Individual T H 17 clones specific for M. tuberculosis were either left resting or were restimulated with plate-bound anti-CD3 and anti-CD28 antibodies for 5 days, after which expression of ID3 , RORC and IL17 was measured by qRT–PCR. Shown are the compiled data of six independent clones, representative of two independent experiments. ( c ) T H 17 cells were sorted ex vivo and transfected with a siRNA against ID3 (siID3) or a negative control (siCTRL). Cells were allowed to recover for 48 h before stimulation with anti-CD3 and anti-CD28 antibodies for another 48 h hours, after which expression of ID3 , RORC and IL17 was measured by qRT–PCR. Representative of at least three independent experiments. ( d ) Ex vivo -isolated T H 17 cells were transfected with a plasmid to force expression of ID3 or with a control plasmid expressing only GFP. Forty-eight hours after transfection, total RNA was extracted and levels of ID3 , RORC and IL17 were assessed by qRT–PCR. Data are representative of at least three independent experiments. Full size image To address whether ID3 induction directly determined the downregulation of RORC and IL17 expression, we transfected T H 17 cells sorted ex vivo from peripheral blood with an siRNA against ID3 (siID3) ( Fig. 6c ). Cells were then stimulated with anti-CD3 and anti-CD28 antibodies for 2 days before RNA extraction and assessment of ID3, RORC and IL17 expression. Upon siRNA-mediated knockdown of ID3 expression, stimulated cells recovered both RORC and IL17 expression ( Fig. 6c ), indicating that ID3 upregulation upon TCR engagement directly led to the downregulation of RORC and IL17 transcription. To further confirm the role of ID3 in regulating RORC expression, we transfected ex vivo- isolated resting T H 17 cells with a plasmid expressing ID3. Transfection efficiency was ~70%, as indicated by the GFP expressed from the same mRNA as ID3. Forty-eight hours after transfection, cells were lysed for RNA extraction. Compared with a GFP-only expression vector (pGFP), cells transfected with the ID3-expressing plasmid (pID3) showed strongly reduced RORC and IL17 expression ( Fig. 6d ), further indicating that ID3 induction repressed these genes in activated T H 17 cells. Sustained ERK phosphorylation in T H 17 cells therefore determines both the threshold of T H 17 cell activation in response to secondary encounters with an antigen, and ID3 induction, thereby leading to the transient loss of IL-17 production observed in recently activated T H 17 cells. Such reduction in cytokine production may represent a cell-intrinsic mechanism aimed at dampening inflammation and tissue damage. T-cell responses must be carefully regulated and resolved to avoid collateral tissue damage and, in some cases, chronic pathology [36] . It is now clear that a complex regulatory network comprising both transcriptional and post-transcriptional components is responsible for the differentiation, maintenance and function of the different T-cell subsets [9] . Here, we showed that given the same TCR specificity, the phenotype acquired by a T cell during the primary response also influences the threshold of activation to a subsequent encounter with the same antigen. Given a similar cytokine environment, each naive T cell has an intrinsic tendency to produce certain types of effector cells in part because of the nature of its unique TCR [37] . Indeed, it is well established that the strength of TCR stimulation determines the capabilities of naive T cells to polarize to specific subsets [6] , [7] . Vice versa, here we showed that the specific phenotype of a memory T cell also determines the threshold of its response to a secondary encounter with the same antigen. In other words, given the same TCR specificity, memory T H 17 cells will be able to respond to lower concentrations of antigen with full-blown activation and proliferation, as compared, for example, with memory T H 2 cells. Such lower threshold of activation in response to a specific antigen may also partially account for the pathogenicity of T H 17 cells in certain autoimmune diseases. The molecular mechanism underlying the enhanced responses in T H 17 cells relies on the sustained ERK phosphorylation observed in memory T H 17 cells compared with other subsets ( Fig. 7 ). ERK phosphorylation is maintained by a self-sustaining, feed-forward loop that includes miR-181a and leads to the reduced expression of ERK-specific phosphatases. Sustained ERK phosphorylation determines on one hand a reduced activation threshold upon re-encounter of a memory T H 17 cell with its cognate antigen, and on the other a transient downregulation of IL-17 production mediated by the induction of the negative regulator ID3. Importantly, as we previously showed [18] , a second pathway converges on the promoters of the RORC and IL17 genes and negatively modulates their expression: indeed, activated T H 17 cells express CD25 (IL-2Rα), thereby becoming responsive to IL-2. IL-2-activated STAT5 competes with phospho-STAT3 for the IL17 promoter and thus negatively impacts on its activation [30] . During priming of naive T cells, the initial cytokine signalling is responsible for the establishment and/or maintenance of higher levels of miR-181a expression specifically in T H 17 cells, with IL-6, IL-1β and TGFβ (but not IL-4 or IL-12) being all able to induce, to various extents, the expression of this miRNA. 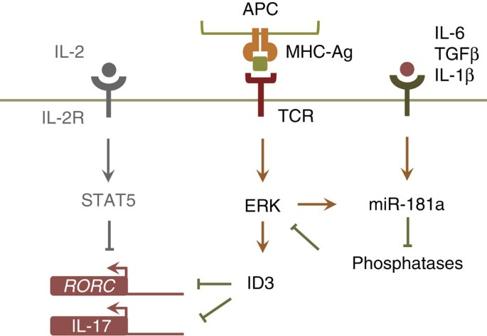Figure 7: Modulation of memory TH17 cell responses by miR-181a and ERK. Non-comprehensive representation of TCR and IL-2 signalling in memory T cells, highlighting the novel findings of this study. ERK phosphorylation is maintained in human memory TH17 cells by miR-181a, which leads to the reduced expression of ERK-specific phosphatases. Initial induction of miR-181a expression upon priming of naive T cells is specifically mediated by cytokines that favour TH17 polarization, such as IL-6, IL-1β and TGFβ. Sustained ERK phosphorylation not only regulates the activation threshold upon TCR triggering in TH17 cells, but it also leads to a transient downregulation of cytokine production mediated by induction of the negative regulator ID3. A previous study showed that a second, IL-2/STAT5-dependent pathway also converges on the promoters of theRORC/IL17genes to negatively modulate their expression (in grey in the figure)18. IL-2 and TCR signalling also lead to the activation of other pathways in addition to the ones shown in this schematic graph. Figure 7: Modulation of memory T H 17 cell responses by miR-181a and ERK. Non-comprehensive representation of TCR and IL-2 signalling in memory T cells, highlighting the novel findings of this study. ERK phosphorylation is maintained in human memory T H 17 cells by miR-181a, which leads to the reduced expression of ERK-specific phosphatases. Initial induction of miR-181a expression upon priming of naive T cells is specifically mediated by cytokines that favour T H 17 polarization, such as IL-6, IL-1β and TGFβ. Sustained ERK phosphorylation not only regulates the activation threshold upon TCR triggering in T H 17 cells, but it also leads to a transient downregulation of cytokine production mediated by induction of the negative regulator ID3. A previous study showed that a second, IL-2/STAT5-dependent pathway also converges on the promoters of the RORC / IL17 genes to negatively modulate their expression (in grey in the figure) [18] . IL-2 and TCR signalling also lead to the activation of other pathways in addition to the ones shown in this schematic graph. Full size image While a handful of miRNAs were already reported to regulate T H 17 cell differentiation [38] , [39] , [40] , [41] , our data showed that miR-181a reduces the threshold of antigenic stimulation for the TCR specifically in T H 17 cells. Dysregulation of miR-181a in immature T cells was already shown to impair both positive and negative thymic selection [11] . Here, we showed that miR-181a has an additional role in regulating TCR sensitivity also in the periphery upon restimulation of memory T H 17 cells. Such reduced threshold of activation of T H 17 cells compared with other T-cell subsets may lead to increased responses to a specific antigen. Of note, miR-181a was recently associated with the susceptibility to develop EAE in rats, showing higher expression in a strain susceptible to EAE compared with an EAE-resistant one [42] , pointing towards a potential role for miR-181a in regulating specific T H 17-cell responses in autoimmunity. The opposing actions of kinases and phosphatases enzymes in the cell determine the level of phosphorylation of a given protein, and the resulting effect of MAPK signalling depends on both the magnitude and duration of kinase activation [23] . The downregulation of phosphatases mediated by miR-181a is likely to be especially critical for the maintenance of the signal over time: indeed, it has been suggested that kinases collectively control signal amplitude, while phosphatases regulate both amplitude and duration [43] . Excessive activation of MAPK is also associated with many autoimmune and inflammatory diseases [44] . Highlighting an important link between TCR signalling and autoimmunity, basal levels of ERK phosphorylation (but not of p38) were shown to be significantly increased in T cells from patients with rheumatoid arthritis, possibly predisposing them to activate autoreactive T cells [45] . In summary, we have shown that given the same TCR specificity, the phenotype acquired by a T cell during the primary response also influences the threshold of activation to a subsequent encounter with the same antigen. Specifically, T H 17 cells appear to acquire increased sensitivity to lower concentrations of antigen, with an underlying molecular mechanism that involves sustained ERK phosphorylation mediated, at least in part, by miR-181a. Moreover, sustained levels of ERK phosphorylation also mediated other features of T H 17 cells, including a transient downmodulation of cytokine production consequence of ID3 induction as well as IL-2 signalling. We speculate that dysregulation of such network regulating T H 17-cell activation and IL-17 production may have important implications in the development of autoimmune diseases. Human T-cell isolation Blood from healthy donors was obtained from the Swiss Blood Donation Center of Basel and Lugano, with informed consent from the Swiss Red Cross. Peripheral blood mononuclear cells were isolated using Ficoll-Paque Plus (GE Healthcare), and CD14 + monocytes and CD4 + T cells were further isolated by positive selection with CD14 and CD4-specific microbeads (Miltenyi Biotec). Naive and memory T-cell subsets were isolated on the basis of the following markers: CD45RA + CD45RO − CCR7 + CD95 − CD25 − CD8 − (naive); CD45RA − CXCR3 + CCR4 − CCR6 − CD25 − CD8 − (enriched in T H 1); CD45RA − CXCR3 − CCR4 + CCR6 − CD25 − CD8 − (enriched in T H 2); CD45RA − CXCR3 − CCR4 + CCR6 + CD25 − CD8 − (enriched in T H 17). In some experiments central memory (T CM ) T H 17 cells were also used, and were separated as CD45RA − CCR7 + CXCR3 − CCR4 + CCR6 + CD25 − CD8 − . Cells were sorted with a FACSAria (BD Biosciences). Where indicated, T-cell subsets were also separated by cytokine secretion assay (Miltenyi Biotec) on the basis of their ability to produce signature cytokines (INFγ for T H 1, IL-4 for T H 2 and IL-17 for T H 17 cells). Cell culture and polarization T cells were cultured in RPMI-1640 medium supplemented with 2 mM glutamine, 1% non-essential amino acids, 1% sodium pyruvate, penicillin (50 U ml −1 ), streptomycin (50 μg ml −1 ) and 5% human serum (Swiss Blood Center). For T-cell cloning, T cells were distributed at 0.5 cells per well in 384-well plates in the presence of IL-2 (500 U ml −1 ), 1 μg ml −1 of phytohaemagglutinin (PHA) as well as 25.000 irradiated (45 Gy) allogeneic feeders (peripheral blood mononuclear cells) per well as previously described [26] . The clones were transferred after 2 weeks to round-bottom 96-well plates and expanded. Antigen-specific T-cell clones were generated from memory T cells as previously described [18] , [26] . Briefly, memory T-cell subsets were labelled with CFSE according to standard protocols; after 5 days of stimulation with antigen-pulsed monocytes (see below), CFSE-negative cell populations were sorted and cloned by limiting dilution, and stimulated with PHA, irradiated allogeneic feeder cells and IL-2. For some clones, the TCR Vβ sequences were obtained following amplification with Vβ-specific primers, and clonotypes bearing identical receptor were identified among different subsets (namely CCR6 − CCR4 + for T H 2 and CCR6 + CCR4 + for T H 17). T-cell stimulation Memory T cells isolated ex vivo were stimulated with plate-bound anti-CD3 (concentrations as indicated in figures, clone TR66) and anti-CD28 (1 μg ml −1 , clone CD28.2) or antigen-pulsed monocytes. Autologous monocytes were pre-incubated for 3 h with whole particles or lysates of C. albicans and irradiated (45 Gy) before co-culture with T cells, as previously described [18] . Briefly, C. albicans conidia were killed by heating at 65 °C for 1 h. Lysate was prepared through repeated sonication cycles of C. albicans suspension (30 cycles, 45 s on, 90 s off on ice), and sterile filtered at 0.22 μm. Protein concentration was determined by Bradford reagent assay (Bio-Rad), and the optimal concentrations of inactivated microorganisms to use in co-culture experiments were determined after titration in proliferation assays using 3 H-thymidine incorporation. T-cell proliferation was measured 2–3 days after initial stimulation, upon addition of 1 mCi ml −1 3 H-thymidine (Perkin Elmer) for 16 h. In some experiments, T-cell clones specific for M. tuberculosis were also used. M. tuberculosis whole-cell lysates were purchased from BEI Resources and used at 5 μg ml −1 . Where indicated, CFSE-labelled memory T cells were stimulated with plate-bound anti-CD3 and anti-CD28 in the presence of increasing concentration of ERK inhibitor (MEK kinase inhibitor, PD98059, Invivogen) and proliferation was measured by CFSE dilution. Mouse colonies All mice were bred and maintained under specific pathogen-free conditions. C57Bl/6 mice were obtained from Harlan (Italy), while TCR MOG 2D2 mice were obtained from V. Kuchroo [25] . Female animals of 6–10 weeks of age were used in all the experiments. The animals were treated in accordance with guidelines of the Swiss Federal Veterinary Office and experiments were approved by the Dipartimento della Sanitàe Socialità of Canton Ticino, authorization number 09-2012. Murine T-cell differentiation For in vitro T-cell differentiation, sorted naive CD4 + CD25 − CD62L-high and CD44-low 2D2 cells [25] were activated with plate-bound anti-CD3 and anti-CD28 (2 μg ml −1 each) in the presence of polarizing cytokines and anti-cytokine antibodies as described [46] , [47] . Briefly, the following polarizing cytokines were added to the cultures: IL-12 (for T H 1 conditions), IL-4 (for T H 2 conditions), IL-6 and TGFβ (for T H 17 conditions). In the non-polarizing ‘Th0’ condition, no cytokines were added to the culture. For in vivo T-cell polarization, 10 5 naive 2D2 cells T cells (CD90.1) were injected in the tail vein of C57Bl/6 mice. The following day, mice were immunized subcutaneously with 150 μg of myelin oligodendrocyte glycoprotein peptide fragment 35–55 (MOG 35–55 ) in the presence of two different adjuvants, complete Freund’s adjuvant (with 4 mg ml −1 of M. tuberculosis H37RA, Difco) or Imject Alum (Pierce Biotechnology). After 6 days, 2D2 cells were recovered from the draining lymph nodes and were restimulated in vitro with bone marrow-derived dendritic cells (matured overnight with 0.5 μg ml −1 of ultrapure Escherichia coli O111-BA LPS, Invivogen) pulsed with increasing concentration of MOG 35–55 peptide. Bone marrow-derived dendritic cells were generated according to a standard protocol [48] using the supernatant of a GM-CSF producing cell line [49] , [50] . Cell proliferation was assessed after 3 days by 3 H-thymidine incorporation assay. RNAi and miRNA transfection For miRNA overexpression and functional ablation, specific oligonucleotides (miR-181a mimic, antagomir and negative scrambled controls) were purchased from ThermoScientific and Exiqon. For RNAi-mediated knockdown of ID3, a previously described siRNA against human ID3 (ref. 51 ) was used (ThermoScientific, Dharmacon). For transfection of miRNAs or siRNAs, 1–2 × 10 6 memory T-cell subsets were transfected with 200 pmol oligonucleotides or controls, using Amaxa Nucleofector reagent (Lonza) and Amaxa electroporator with program U-14 following manufacturer’s instructions. In preliminary experiments, efficiency of transfection was assessed using a fluorescent oligonucleotide (siGLO, ThermoScientific). After 48 h from transfection, T cells were stimulated with plate-bound anti-CD3 and anti-CD28 or antigen-pulsed monocytes. The proliferation rate was measured after 3 days on addition of 1 mCi ml −1 3 H-thymidine for 16 h. Plasmids The full-length cDNA for human ID3 was purchased from OriGene and subcloned into a mammalian expression vector using common cloning techniques. Memory T-cell subsets (1–2 × 10 6 ) were transfected with 1 μg of plasmid using Amaxa (program U-14). Intracellular staining To assess cytokine production, cells were stimulated for 5 h with PMA (200 nM) and ionomycin (1 μg ml −1 ) in the presence of 10 μg ml −1 brefeldin A (all from Sigma-Aldrich) for the final 2.5 h of culture before fixation and permeabilization with Cytofix/Cytoperm (BD Biosciences), according to manufacturer’s instructions. Cells were then stained with anti-IL-17, anti-IFNγ and anti-IL-4 antibodies conjugated to different fluorochromes, and were acquired on a FACSCanto (BD Bioscience). Flow cytometry data were analysed with FlowJo (Tree Star). For intracellular detection of phosphorylated ERK (pERK), cells were stimulated with plate-bound anti-CD3 and anti-CD28 for the indicated times, prior fixation with 3.7% formaldehyde and permeabilization with 90% methanol. Staining was performed with a 1:200 dilution of a phospho-specific-p44/42 MAPK (Erk1/2) (Thr202/Tyr204) (Cell Signaling; cat no. 4377S). RNA extraction and quantitative PCR with reverse transcription (qRT–PCR) Total RNA was extracted using TRIzol reagent (Invitrogen) according to manufacturer’s instructions. Random hexamer primers and a reverse transcriptase kit (Stratagene) were used for cDNA synthesis. Transcripts were quantified by qRT–PCR on an ABI PRISM 7900HT with predesigned TaqMan Gene Expression Assays and reagents (Applied Biosystems). TaqMan assays were as follows: IL17A (Hs99999082), RORC (Hs01076122_m1), ID3 (Hs00171409_m1), DUSP5 (Hs00244839_m1), PTPN11 (Hs00743983_s1), DUSP6 (Hs04329643_s1). To analyse miRNA expression levels, qRT–PCR was performed using a miRNA reverse transcription kit and TaqMan miRNA assays from Applied Biosystems, following manufacturer’s instructions. Expression of target genes and miRNAs were normalized to 18S ribosomal RNA and RNU48, respectively. For data analysis, the ΔΔCt method was used [52] . TCR Vβ analysis and sequencing were performed exactly as described [24] , [27] . Statistical analysis Statistical analysis was performed with the Prism software (GraphPad). Data are represented as mean±s.e.m. or s.d., and significance was assessed by paired or unpaired Student’s t -test, two-tailed. How to cite this article: Mele, F. et al. ERK phosphorylation and miR-181a expression modulate activation of human memory T H 17 cells. Nat. Commun. 6:6431 doi: 10.1038/ncomms7431 (2015).